Laminar activity in the hippocampus and entorhinal cortex related to novelty and episodic encoding The ability to form long-term memories for novel events depends on information processing within the hippocampus (HC) and entorhinal cortex (EC). The HC–EC circuitry shows a quantitative segregation of anatomical directionality into different neuronal layers. Whereas superficial EC layers mainly project to dentate gyrus (DG), CA3 and apical CA1 layers, HC output is primarily sent from pyramidal CA1 layers and subiculum to deep EC layers. Here we utilize this directionality information by measuring encoding activity within HC/EC subregions with 7 T high resolution functional magnetic resonance imaging (fMRI). Multivariate Bayes decoding within HC/EC subregions shows that processing of novel information most strongly engages the input structures (superficial EC and DG/CA2–3), whereas subsequent memory is more dependent on activation of output regions (deep EC and pyramidal CA1). This suggests that while novelty processing is strongly related to HC–EC input pathways, the memory fate of a novel stimulus depends more on HC–EC output. There is now converging evidence that the hippocampus (HC) and the adjacent entorhinal cortex (EC) are required to successfully encode detailed information about novel events into long-term memory (for reviews, see refs 1 , 2 ). Bilateral lesions of these regions lead to a long-term memory impairment that is characterized by an inability to recollect details about novel events [2] , [3] , [4] . The HC consists of the HC proper with subfields CA3, CA2 and CA1, the dentate gyrus (DG) and the subiculum. Although substantial progress has been made towards demonstrating the involvement of HC subfields and the EC in memory encoding in human imaging studies (for reviews, see refs 5 , 6 ), an understanding of circuit-level mechanisms underlying encoding operations in the human HC–EC has not been possible to date. Components of the HC are linked to the EC through anatomically well-characterized circuits (for a review, see ref. 7 ). The major pathway from the EC to HC is the perforant path, which projects to DG and CA3 and from there to the stratum radiatum and stratum lacunosum-moleculare (SRLM) of the CA1 region (indirect pathway; see, for example, ref. 8 ). The SRLM of CA1 also receives a direct perforant pathway projection from EC. Intriguingly, input and output operations are quantitatively segregated into different laminae of the EC and HC subfields. That is, the more superficial layers II and III of EC project to DG/CA3 and the apical layer of CA1, respectively, whereas HC output reaches primarily the deep entorhinal layers V, VI (see, for example, refs 7 , 9 , 10 ). The HC output to EC originates in CA1 from layers containing the pyramidal cells, stratum pyramidale and its deepest layer, stratum oriens (containing a mixture of the axons of the pyramidal cells, afferent fibres and interneurons), as well as the subiculum. Although this layer-specific organization of HC inputs and outputs within EC is not exclusive (for example, deep EC layers also contribute to input into the HC [11] , [12] ) and there are a number of published exceptions, in quantitative terms this pattern is dominant [7] . In our study, we divided the EC into three equally sized subregions: superficial, middle and deep. Although the anatomical layering of the EC could not be identified on our MR images, previous ultra-high-resolution ex vivo MRI studies [13] , [14] suggest that our superficial EC subregion very likely corresponds to EC input layers (covering layer II and probably parts of layer III), whereas our deep EC subregion likely covers the output layers of the EC (V and VI). The HC–EC circuitry is at the top of a visual processing hierarchy [2] , [15] and receives inputs about object representations from perirhinal cortex (PRC) and space representations from parahippocampal cortex (PHC). These inputs are likely to remain segregated in EC until they converge to object-in-space scene representations in the HC [2] , [16] , [17] , [18] . FMRI studies of scene processing have consistently observed ‘novelty responses’ (stronger fMRI activation for novel as compared with familiar stimuli) in these regions [19] , [20] . Using subfield and layer-specific fMRI, we were now able to assess the distribution of novelty responses for scenes within input and output regions of the HC–EC circuitry. For the following reasons, novelty responses could dominate in the input structures of the circuitry. The superficial (input) layers of EC should show novelty responses because these already receive afferent novelty signals from object and space processing pathways. On the basis of previous human fMRI data showing higher activation for novel than repeated objects [21] , we would also expect novelty responses in DG/CA3, which probably rest on an automatic representational orthogonalization process (‘pattern separation’) in the DG that reduces the probability of interference in memory (for example, ref. 22 ). Previous studies in rodents [23] , [24] and fMRI studies in humans [21] have also shown activation of CA1 during novel experiences. These novelty responses are predicted, for instance, by comparator models, which posit that comparison of input from the EC to CA1 with input that CA1 receives from CA3 aids the assessment of novelty [25] . According to comparator models [25] , novelty should be associated with correlated activity of the superficial entorhinal layers with DG/CA3, as well as with the SRLM of CA1, the latter being compatible with input from the EC to CA1 via the perforant path. In addition to investigating which regions show novelty responses, we assessed whether activation in the same regions also predicted the ability to subsequently recollect the novel scenes. An anatomical overlap between novelty and subsequent recollection would indicate that the functional strength of stimulus novelty in a given region is related to successful memory. For instance, when the subject is exposed to a series of novel scene images, effective pattern separation in DG/CA3 would prevent that incidental similarities between different scenes reduce novelty responses and at the same time improve subsequent memory (see, for example, ref. 21 ). We also assessed the alternative possibility that the ability to later remember information is influenced by hippocampal mechanisms that do not depend on the strength of the stimulus novelty response. For instance, the aforementioned CA1 comparator process has also been hypothesized to incorporate predictions about the sequence of stimuli [26] (for example, if several successive stimuli belong to one of two categories, a category change may be predicted), a process which could generate match/mismatch output signals in CA1 that influence memory independent of stimulus novelty. Furthermore, complementary systems learning models [27] , [28] postulate that cooperation between CA1 and the output (deep) layers of EC is important for recollection because it allows pattern-separated CA3 representations to be decoded into a format that can be fed back to the cortex [27] , [29] and the success of this decoding could potentially also be independent of novelty. According to this possibility, and in contrast to stimulus novelty, activity predicting successful memory would, therefore, be dominant in the output structures of the HC–EC circuitry (including pyramidal layers of CA1 and deep EC). Thus, the HC would produce an output only for some of the novel information that it receives, namely those that can be later remembered. In order to address these hypotheses, it is necessary to measure activity of the entire HC–EC network with a spatial resolution that is high enough to segregate activity at a laminar level. Thus far, high resolution fMRI studies of the human medial temporal lobe (MTL) have been largely conducted using scanners with field strengths of 3 T, which permit a resolution of up to 1.5 × 1.5 × 1.5 mm (corresponding to a volume of 3.375 mm 3 ). Although this resolution allowed isolating activity in hippocampal subfields and EC (for example, refs 5 , 6 , 21 ), selective recordings from laminae of the entire circuitry have not been reported yet. To measure layer-specific activation in the HC–EC circuitry, we used fMRI at an ultra-high field of 7 T (for a recent feasibility study of 7 T fMRI of the MTL, see ref. 30 ) with a functional resolution of 0.8 × 0.8 × 0.8 mm (corresponding to a volume of 0.51 mm 3 ) and hence more than 6.6 times higher than previous high resolution studies at 3 T. The feasibility of detecting layer-specific blood oxygenation level dependent (BOLD) activation in the visual cortex has been demonstrated already in previous studies with cats, monkeys and humans (see, for example, refs 31 , 32 , 33 ). Furthermore, it has been shown that there exist laminar differences in BOLD, cerebral blood volume and cerebral blood flow responses between stimulated and unstimulated cortical regions, indicating layer-specific differences in the neurovascular coupling [33] . Although the underlying hemodynamic processes are not fully resolved, laminar differences in the fMRI responses open up the possibility to study cortical processing at the level of layers. In the present study, fMRI data were recorded while healthy young adults engaged in an incidental encoding task with novel and prefamiliarized images of scenes. Recognition memory for the novel scenes was later tested outside of the scanner via memory confidence judgments that allowed us to quantify recollection- and familiarity-based memory (see, for example, refs 28 , 34 ). To address the aforementioned hypotheses regarding novelty and subsequent memory, we were particularly interested in differences of activity between entorhinal input and output regions and between hippocampal subfields and layers. Therefore, we used a Bayesian decoding approach (Multivariate Bayes (MVB) [35] ) that is suited to decide, based on fMRI activity in individual subjects and without the need for spatial normalization, which region provides the best explanation of a given cognitive process (that is, novelty or subsequent memory). MVB decoding revealed that processing of novel scenes was best predicted by activation in the input structures (superficial EC and DG/CA2–3), whereas subsequent memory was best explained by activation of output regions (deep EC and pyramidal CA1). Furthermore, later recollection performance across subjects was predicted by the activation strength in CA1 pyramidal (output) layers. Functional connectivity analyses showed that activity in pyramidal layers of CA1 and deep EC regions was correlated during successful encoding. This suggests that while novelty processing is strongly related to HC–EC input pathways, the memory fate of a novel stimulus depends more on HC–EC output. Overview of data analyses First, we performed group-level analyses (one-sample t -tests), which require smoothing and normalization of the functional data in order to show that EC and HC regions were significantly activated across subjects and furthermore, to make our data comparable and relatable to the previous fMRI literature. In a second step, we used MVB to evaluate functional differences between EC and HC layers/subregions with maximum spatial precision by using individual unsmoothed data. Finally, we analysed if the strength of subfield- or layer-specific activity in the HC–EC circuitry was predictive for later recognition performance across subjects and furthermore if subregion-specific activation in the EC was functionally correlated with activation of the HC. All analyses were performed on bilateral data. Group activation in hippocampal and entorhinal subregions During the fMRI session, subjects performed an incidental visual-encoding paradigm on images of scenes and repetitions of one prefamiliarized image. In a later recognition task, images presented during the fMRI session were intermixed with distractor pictures and memory was tested on a five-point confidence rating scale. Two types of contrasts were analysed. First, activations due to stimulus novelty (‘novelty’; Fig. 1a ) were measured by comparing all new images with the repetitions of the one familiar image. Second, differences in activity due to later memory (difference due to memory, ‘DM’; Fig. 1b ) for the novel items were assessed by contrasting later recognized stimuli with later forgotten items. 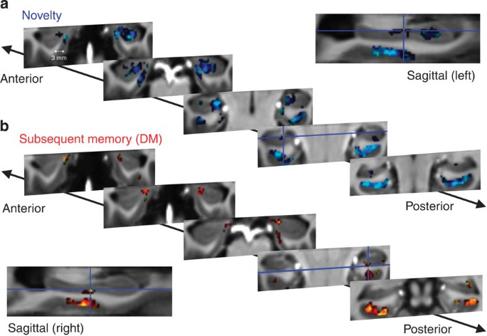Figure 1: Novelty processing and successful memory encoding elicit a distinct activity pattern in hippocampal and parahippocampal subregions. Group activity for (a) novelty and (b) successful encoding (difference due to memory, ‘DM’), overlaid on the group-specific T1 template (with same resolution as functional images: 0.8 mm isotropic voxels) after ROI-based diffeomorphic registration with ANTS. Group activation is illustrated on five coronal sample slices for two different smoothing kernels. EPIs were initially smoothed with 1.5 mm (<2 × voxel size, bright colours: cyan and yellow), which allows for higher anatomical precision at the cost of lower sensitivity. Furthermore, the analyses were repeated with a 2.4 mm FWHM (=3 × voxel size, dark colours: blue and red) to increase sensitivity and demonstrate reliability of activation. For both contrasts, there was significant activation in the EC (mostly medial). In the hippocampus, novelty-related activation was most prominent in the head with peak activation in CA2/3-DG and presubiculum. For successful encoding, hippocampal activation was found in CA1 pyramidal layers (slice 4, cluster right to cross-hairs) and subiculum (head & body, see cross-hairs) and a small cluster in CA2/3-DG (posterior body). Activation maps were thresholded atPvoxel level<0.005≈T>2.9;k1.5 mm≥15 voxels andk2.4 mm≥25 voxels (N=19). Figure 1: Novelty processing and successful memory encoding elicit a distinct activity pattern in hippocampal and parahippocampal subregions. Group activity for ( a ) novelty and ( b ) successful encoding (difference due to memory, ‘DM’), overlaid on the group-specific T1 template (with same resolution as functional images: 0.8 mm isotropic voxels) after ROI-based diffeomorphic registration with ANTS. Group activation is illustrated on five coronal sample slices for two different smoothing kernels. EPIs were initially smoothed with 1.5 mm (<2 × voxel size, bright colours: cyan and yellow), which allows for higher anatomical precision at the cost of lower sensitivity. Furthermore, the analyses were repeated with a 2.4 mm FWHM (=3 × voxel size, dark colours: blue and red) to increase sensitivity and demonstrate reliability of activation. For both contrasts, there was significant activation in the EC (mostly medial). In the hippocampus, novelty-related activation was most prominent in the head with peak activation in CA2/3-DG and presubiculum. For successful encoding, hippocampal activation was found in CA1 pyramidal layers (slice 4, cluster right to cross-hairs) and subiculum (head & body, see cross-hairs) and a small cluster in CA2/3-DG (posterior body). Activation maps were thresholded at P voxel level <0.005≈T>2.9; k 1.5 mm ≥15 voxels and k 2.4 mm ≥25 voxels ( N =19). Full size image To assess which hippocampal and entorhinal subregions were significantly activated across subjects, we calculated second-level group activation maps after regions of interest (ROI)-based alignment with ANTS [36] (Advanced Normalization Tools; see Methods and Supplementary Fig. 1 ). Functional data were smoothed with two different smoothing kernels (full-width half-maximum (FWHM): 1.5 mm < 2 × voxel size and 2.4 mm=3 × voxel size) to demonstrate the reliability of activation patterns across different levels of smoothing and to assess activations from the perspectives of either higher specificity (smoothing with 1.5 mm) or higher sensitivity (smoothing with 2.4 mm). A summary of activated EC/HC regions is shown in Tables 1 and 2 and Fig. 1 , in which activation maps for the low smoothing kernel (light colours) are overlaid on the higher smoothing results maps (dark colours). Table 1 Novelty-related group activation after ROI-based alignment. 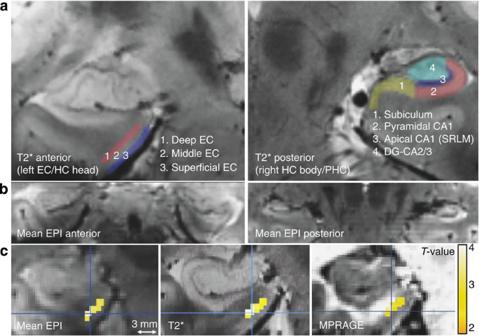Figure 2: Segmentation scheme of entorhinal and hippocampal subregions and layer-specific sample activation. (a) Single-subject high resolution T2* image (resolution: 0.33 mm2in-plane, 1.5 mm slice thickness) with overlaid entorhinal (EC; left panel) and hippocampal (HC; right panel) ROIs on two coronal slices. ROIs were manually segmented on the individual T2* images and coregistered to the mean EPIs. The EC was equally divided into three regions: superficial, middle and deep. The CA1 region in the hippocampal body was subdivided into apical (Nr. 3) and pyramidal regions (Nr. 2). Note that the apical dendritic layer of CA1 (‘SRLM’) is well visible as a dark band on T2-weighted images. (b) Individual mean functional MR image (EPI, resolution: 0.8 mm3) showing anterior MTL regions (EC, PRC and hippocampal head; left panel) and more posterior MTL regions (PHC and hippocampal body; right panel). (c) Single-subject (peak) activation due to memory (DM, or successful encoding) overlaid on the individual mean EPI and the coregistered T2* and MPRAGE image (smoothing: 1.5 mm,Pvoxel level<0.01,k≥10 voxels). This demonstrates that activation can be confined to deep (vs superficial subregions) of the EC. For single-subject peak activation see alsoSupplementary Fig. 2. Full size table Table 2 Subsequent memory (‘DM’)-related group activity after ROI-based alignment. Full size table For both contrasts, second-level group analysis yielded most prominent activation in medial EC and anterior HC. For novelty, strongest hippocampal activity was found in DG/CA2–3 and subiculum/presubiculum, especially in the hippocampal head. Several activity clusters were also located in CA1. With regard to successful encoding activity for the new stimuli (DM contrast), strongest HC activity was found in the pyramidal layer of CA1 (close to the outer hippocampal border; see Fig. 1b and Table 2 ). Furthermore, several clusters were located in the head (medial CA1 and subiculum/presubiculum). Although some reported clusters did not survive multiple comparison correction for the low smoothing kernel (FWHM: 1.5 mm), we could demonstrate reliability of activation by increasing sensitivity with a higher smoothing kernel (FWHM: 2.4 mm). Furthermore, we did not find any activation in HC or EC when testing for the inverse novelty contrast (familiarity-related activity; P voxel level <0.005: no cluster>1 voxel) or the inverse DM contrast (higher activation for subsequently forgotten items; P voxel level <0.005: no cluster>4 voxels). In summary, the above univariate second-level analyses revealed significant activations in EC and specific HC subfields. MVB decoding of novelty and subsequent memory To measure laminar activity in the EC, we subdivided the grey matter of the EC into three equally sized portions (superficial, middle and deep; see Fig. 2a for segmentation scheme of ROIs). Kerchner et al. [37] reported the thickness of the human EC to be 2.7 mm, while in Fischl et al. [38] the mean thickness was 3.1 mm. With an isotropic voxel size of 0.8 mm, and after segmenting the EC into three sections, we obtained EC subregions with ~1 mm thickness and were thus able to measure activity selectively in superficial and deep regions of the EC (see Fig. 2c and Supplementary Fig. 2 for single-subject peak activation). Furthermore, we traced the apical dendritic layer (SRLM) of the CA1 region, which is visible on T2*-weighted images [37] and can be distinguished from the rest of CA1 (stratum pyramidale, stratum oriens, see Fig. 2a ). Although the SRLM is slightly thinner than our voxel size (ca. 0.68 mm (ref. 37 )), its segmentation allows us to make a first step towards separating laminar activity in pyramidal from apical CA1 regions (and also from activity in DG/CA3) and thus, to analyse activation related to hippocampal output pathways. Figure 2: Segmentation scheme of entorhinal and hippocampal subregions and layer-specific sample activation. ( a ) Single-subject high resolution T2* image (resolution: 0.33 mm 2 in-plane, 1.5 mm slice thickness) with overlaid entorhinal (EC; left panel) and hippocampal (HC; right panel) ROIs on two coronal slices. ROIs were manually segmented on the individual T2* images and coregistered to the mean EPIs. The EC was equally divided into three regions: superficial, middle and deep. The CA1 region in the hippocampal body was subdivided into apical (Nr. 3) and pyramidal regions (Nr. 2). Note that the apical dendritic layer of CA1 (‘SRLM’) is well visible as a dark band on T2-weighted images. ( b ) Individual mean functional MR image (EPI, resolution: 0.8 mm 3 ) showing anterior MTL regions (EC, PRC and hippocampal head; left panel) and more posterior MTL regions (PHC and hippocampal body; right panel). ( c ) Single-subject (peak) activation due to memory (DM, or successful encoding) overlaid on the individual mean EPI and the coregistered T2* and MPRAGE image (smoothing: 1.5 mm, P voxel level <0.01, k ≥10 voxels). This demonstrates that activation can be confined to deep (vs superficial subregions) of the EC. For single-subject peak activation see also Supplementary Fig. 2 . Full size image Since these layers are difficult to visually identify in the DG, this region, as well as CA3 and subiculum were manually segmented as subfields without layer-specific compartmentalization. Furthermore, segmentation of HC layers and subfields was only performed in the body, where borders could be precisely identified and not in the hippocampal head (see Methods section for details). To test if layers or subfields in the EC or HC showed differential responses to novelty and subsequent memory, we used a model comparison approach based on a multivariate decoding scheme. Specifically, we performed MVB decoding analyses [35] to evaluate whether novel trials (vs familiar trials) or remembered trials (vs forgotten trials) can be better predicted from distributed activity in one subregion compared with another. This method allows the use of individual (not normalized) functional data to compute the log evidences for each subject-specific anatomical mask and is particularly suited to make comparisons across regions. For the second-level analysis, we chose random-effects Bayesian model selection (BMS [39] ). Posterior model probabilities are compared by deriving the exceedance probability (xp) of each model, that is, the probability that this model is more probable than any other model tested. MVB analyses were performed on bilateral data. First, we used MVB to test whether novelty or subsequent memory (DM) can be better predicted from activity in superficial EC than deep EC (or vice versa). In addition, we defined a mask in the anterior brainstem for each subject, which served as a control region (with the same number of voxels as in the individual EC ROIs) to test if our results were specific to EC subregions and would not emerge in regions not motivated by our hypothesis. This control region was included in all our subsequent MVB analyses, that is, in the same way as for our ROI. Second-level random effects analyses showed that novelty was best predicted from activity in superficial EC compared with deep EC (xp: superficial EC=100.0%, deep EC=0%, brainstem=0%; see Fig. 3a ; with 18 of our 20 subjects showing highest log evidence for superficial EC). In contrast, subsequent memory was best predicted from activity in deep EC compared with superficial EC (xp: superficial EC=2.1%, deep EC=97.8%, brainstem=0.1%; see Fig. 3b ; with 15 subjects showing highest log evidence for deep EC). These results demonstrate the differential engagement of separate EC subregions during novelty processing and successful memory encoding. Furthermore, the log evidences for predicting novelty and subsequent memory, respectively, from activity in the brainstem control region did not differ between both contrasts ( P >0.50) and were also much lower than the log evidences for all EC subregions (see Fig. 3 ). Please note that superficial and deep EC ROIs did not differ in size across subjects ( P >0.19). Univariate analyses confirmed the findings from MVB decoding and showed that the number of activated voxels was higher in superficial EC subregions during novelty processing and vice versa in the deep EC subregions during successful encoding ( Supplementary Fig. 3a and Supplementary Note 1 ). 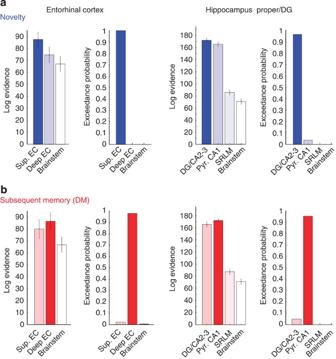Figure 3: Bayesian model comparisons for decoding of novelty and subsequent memory in entorhinal and hippocampal layers/subregions. MVB decoding was used to test whether novelty or subsequent memory (‘DM’) can be better predicted from activity in one region than another. The method allows use of the individual (not normalized, not smoothed) functional data to compute the log evidences for each subject-specific anatomical mask (N=20). The relative probability of one model (subregion) over any other model tested is expressed in terms of the exceedance probability (xp) based on random-effects BMS. As control region, the anterior brainstem was included in all analyses. (a) Novelty: Novel trials were detected with highest probability from activity in superficial (‘input’) subregions within the EC (xp: superficial EC=100.0%, deep EC=0%, brainstem=0%) and from DG/CA2–3 within the hippocampus proper/DG (xp: DG/CA2–3=96.3%, pyr. CA1=3.7, SRLM=0.0%, brainstem =0). (b) DM: In contrast, subsequent memory was better decoded from deep (‘output’) subregions within the EC (xp: superficial EC=2.1%, deep EC=97.8%, brainstem=0.1%) and pyramidal CA1 (‘output’) layers within HC proper/DG (xp: DG/CA2–3=4.8%, pyr. CA1=95.2, SRLM=0.0%, brainstem =0.0). Please note that hippocampal analyses were restricted to the hippocampal body where subfields and CA1 apical (‘SRLM’) and pyramidal layers could be reliably differentiated. Error bars denote s.e.m. Figure 3: Bayesian model comparisons for decoding of novelty and subsequent memory in entorhinal and hippocampal layers/subregions. MVB decoding was used to test whether novelty or subsequent memory (‘DM’) can be better predicted from activity in one region than another. The method allows use of the individual (not normalized, not smoothed) functional data to compute the log evidences for each subject-specific anatomical mask ( N =20). The relative probability of one model (subregion) over any other model tested is expressed in terms of the exceedance probability (xp) based on random-effects BMS. As control region, the anterior brainstem was included in all analyses. ( a ) Novelty: Novel trials were detected with highest probability from activity in superficial (‘input’) subregions within the EC (xp: superficial EC=100.0%, deep EC=0%, brainstem=0%) and from DG/CA2–3 within the hippocampus proper/DG (xp: DG/CA2–3=96.3%, pyr. CA1=3.7, SRLM=0.0%, brainstem =0). ( b ) DM: In contrast, subsequent memory was better decoded from deep (‘output’) subregions within the EC (xp: superficial EC=2.1%, deep EC=97.8%, brainstem=0.1%) and pyramidal CA1 (‘output’) layers within HC proper/DG (xp: DG/CA2–3=4.8%, pyr. CA1=95.2, SRLM=0.0%, brainstem =0.0). Please note that hippocampal analyses were restricted to the hippocampal body where subfields and CA1 apical (‘SRLM’) and pyramidal layers could be reliably differentiated. Error bars denote s.e.m. Full size image To investigate whether HC subfields or layers show differential responses to novelty and subsequent memory, we performed additional bilateral MVB analyses for the HC proper and the DG (within the hippocampal body where layers and subfields could be clearly defined). Bayesian model comparison showed that novel trials were best explained in terms of DG/CA2–3 activity (xp: DG/CA2–3=96.3%, pyr. CA1=3.7, SRLM=0.0%, brainstem=0; see Fig. 3a ; in 14 subjects the log evidence was highest for DG/CA2–3). In contrast, subsequent memory could be best decoded from pyramidal layers of CA1 compared with other hippocampal subregions (xp: DG/CA2–3=4.8%, pyr. CA1=95.2, SRLM=0.0%, brainstem=0.0; see Fig. 3b ; in 14 subjects the log evidence was highest for pyr. CA1). Please note that DG/CA2–3 and pyramidal CA1 layers did not differ in size across subjects ( P >0.6). However, the SRLM ROI was significantly smaller than the other subregions ( P <0.01) and thus contained a significantly lower number of voxels (=predictors), which might explain the low values in log evidence (compared with DG-CA2/3 and pyramidal CA1). The same pattern of differential activation of DG/CA2–3 and pyramidal CA1 regions was also apparent at the univariate level ( Supplementary Fig. 3b ). Correlations of encoding activity with memory performance Our aforementioned decoding analysis using MVB and subsequent model comparison revealed that within the HC proper/DG, subsequent memory was best explained in terms of activation in pyramidal layers of CA1. To specifically test if activation strength in this region was also correlated with later memory performance across subjects, we extracted the effect size (contrast estimate from the GLM) for all voxels within the anatomically defined pyramidal CA1 ROI and computed its average across voxels. This was done at the single-subject level using the non-normalized and non-smoothed individual first-level DM-maps (see Methods section for details). We found significant correlations of successful encoding (DM) activity in pyramidal CA1 layers with high confidence corrected hit rates (Pearson’s correlation, two-tailed, P =0.014; R =0.54; see Fig. 4a ) and recollection estimates ( P =0.025; R =0.50; see Fig. 4a ). In other words, later recollection across subjects was predicted by activation strength in the pyramidal (output) layers of CA1. 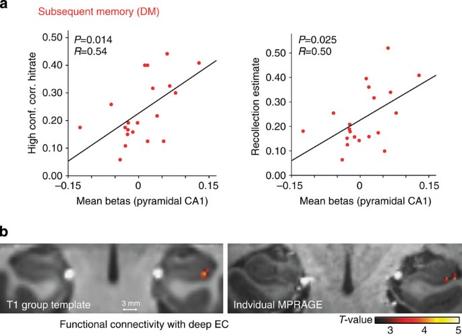Figure 4: Successful encoding activity in pyramidal layers of CA1 predicts later memory and is correlated with activation in deep EC regions. (a) High confidence recognition and recollection estimates in the subsequent memory test were correlated with successful encoding activity strength in the pyramidal (‘output’) layers of CA1 across subjects (N=20). Activation strength is defined as the mean contrast estimate (weighted betas for DM contrast) of all voxels in our anatomically defined ROI (pyramidal CA1). Betas were extracted from the individual unnormalized and unsmoothed functional data using subject-specific anatomical masks. (b) Functional connectivity analyses (PPI) yielded significant functional coupling of deep EC regions (seed) with pyramidal layers of CA1 during successful encoding (Pvoxel level<0.005:k=26 voxels, alpha<0.05,N=19). Group results are depicted on the T1-group template after normalization with ANTS (left). In addition, results are illustrated for one sample subject on the individual MPRAGE (right). Figure 4: Successful encoding activity in pyramidal layers of CA1 predicts later memory and is correlated with activation in deep EC regions. ( a ) High confidence recognition and recollection estimates in the subsequent memory test were correlated with successful encoding activity strength in the pyramidal (‘output’) layers of CA1 across subjects ( N =20). Activation strength is defined as the mean contrast estimate (weighted betas for DM contrast) of all voxels in our anatomically defined ROI (pyramidal CA1). Betas were extracted from the individual unnormalized and unsmoothed functional data using subject-specific anatomical masks. ( b ) Functional connectivity analyses (PPI) yielded significant functional coupling of deep EC regions (seed) with pyramidal layers of CA1 during successful encoding ( P voxel level <0.005: k =26 voxels, alpha<0.05, N =19). Group results are depicted on the T1-group template after normalization with ANTS (left). In addition, results are illustrated for one sample subject on the individual MPRAGE (right). Full size image Although this analysis for the CA1 pyramidal layers was specifically motivated by the MVB results, we note, for completeness, that there were no significant correlations with later memory performance for any other subregion. Except for a trend correlation between contrast estimates in the PHC and familiarity estimates ( P =0.071), all other P values were >0.1. Layer-specific functional connectivity of the EC The above MVB decoding results show that processing of a novel stimulus was best explained in terms of activity in superficial EC, whereas subsequent memory was predicted with highest probability from deep EC. To test whether novelty-related activation in superficial EC correlated with activity in DG/CA2–3 and/or SRLM compatible with input from the EC to the HC, we examined the context-specific coupling of this layer (cf. a psychophysiological interaction (PPI) analysis). For this analysis, individual superficial EC ROIs were used as seed regions. Furthermore, we wanted to test whether successful encoding activity (DM) in deep EC was coupled to activation in pyramidal layers of CA1 and/or subiculum. To that end, we took deep EC ROIs as seeds for the PPI analysis based on successful encoding activity. Connectivity analyses were performed at the single-subject level to ensure the highest anatomical precision. Second-level group analysis (after ROI-based registration with ANTS) of PPI results maps revealed those regions that showed significant context-specific coupling with the seed regions across subjects. Second-level analyses yielded strongest functional connectivity of superficial EC with right anterior DG/CA2–3 (for P voxel level <0.005: k =10 voxels, no other cluster >3 voxels) during novelty processing. However, this cluster would not survive correction for multiple comparisons. For deep EC, strongest functional coupling during successful memory encoding was found with pyramidal layers of right CA1 (for P voxel level <0.005: k =26 voxels, alpha <0.05; see Fig. 4b ). PPI (control) analyses using superficial EC ROIs as seed regions in the DM contrast and deep EC ROIs as seed regions in the novelty contrast did not reveal significant connectivity with any region in the HC ( P voxel level <0.005, no cluster >5 voxels). Comparison between BOLD characteristics of HC and EC Finally, we analysed if there were systematic differences between the BOLD responses in HC and EC. To compare hemodynamic response functions between both regions, we used SPM8 (‘Hemodynamics’; see ref. 40 for details) to estimate hemodynamic model parameters across subjects ( N =20). T -tests on these parameters (feedback, transit time, exponent, resting oxygen extraction and log signal ratio) showed that under the power which our sample size affords, one cannot detect a significant difference in these hemodynamic parameters between regions (all P corr >0.32). This makes it unlikely that the other analyses in the present study are confounded by regional differences in the hemodynamic response function. We used 7 T high resolution fMRI to measure encoding activity in subregions/layers of the EC and of the HC. To compare activation between regions, we chose a Bayesian decoding approach (MVB) that is particularly suited to evaluate competing hypotheses about which anatomical structure hosts a particular cognitive process [35] , [41] . We were able to show differential activation of entorhinal input and output regions with respect to novelty processing and successful memory encoding. Using MVB decoding, we found that novel trials were best predicted from activity in the input regions within the EC and from DG/CA2–3 within the HC proper/DG ( Fig. 3a ; see also Supplementary Fig. 3a for ROI-specific univariate results). Furthermore, we have preliminary evidence that activation in superficial EC is specifically correlated with activity in DG/CA2–3. These observations suggest that the input from EC to the HC is related to novelty because the superficial regions of EC are quantitatively more strongly an origin of input to the HC than being a target of output from the HC. Hence, our data provide combined functional and anatomical evidence that perforant pathway input from EC to the HC is related to novelty processing as predicted by theory [25] . Lesion studies in rats have indicated that the DG–CA3 network plays a key role in processing novel spatial information [42] , which is in line with our results that novelty processing most strongly engaged the DG/CA2–3 subregion. By testing subsequent recognition memory performance for the novel items, we were also able to determine which subfields and layers were related to subsequent memory. Later remembering was better predicted by activity in deep than superficial EC ( Fig. 3b ; see also Supplementary Fig. 3b for ROI-specific univariate results). Regarding the HC proper and DG, subsequent memory was explained in terms of activation in pyramidal CA1 layers. Furthermore, activation strength in the pyramidal layers of CA1 was predictive for later high confidence recognition/recollection performance across subjects ( Fig. 4a ). Finally, our functional connectivity results showed that DM-related responses in deep EC were most strongly correlated with activation of pyramidal CA1 layers ( Fig. 4b ). Our deep EC ROI very likely covered the entorhinal layers V and VI. These deep entorhinal layers are more strongly a target of output from the HC (that mostly arises from the pyramidal layers of CA1 and subiculum) than providing input to HC. Therefore, these findings suggest that the ability to later recollect the exposure to a novel item is more related to the results of intrinsic computations within HC and EC and their output-level activity (during encoding) than the strength of activity driving input to the HC from EC. Multivariate Bayesian decoding within EC regions related activity in superficial (input) and deep (output) EC to novelty and subsequent memory, respectively. Previous studies in primary sensory areas have shown that draining venous blood might affect the signal of deep and superficial layers differently (draining vein effect) with a bias towards responses from superficial layers (see, for example, refs 31 , 32 , 43 ). However, systematic differences of BOLD responses between the layers cannot explain our findings of an inverse activation pattern for the DM contrast compared with novelty in superficial vs deep EC. Although the BOLD signal from superficial regions might contain a hemodynamic contribution from the deep regions, this only makes the inference about what is encoded by superficial regions more conservative. In other words, finding that BOLD signal from the superficial EC encodes novelty despite a putative confounding hemodynamic influence from the deep EC speaks to the robustness of our results. There is converging evidence that novelty encoding in the HC should primarily support the ability to later recollect associative information about the context and episodic details with which a novel item was encountered, such as time and location [2] , [3] , [44] . In contrast, a mere increase in familiarity recognition due to previous exposure can be preserved even after bilateral hippocampal lesions [3] , [44] , suggesting that familiarity per se does not critically depend on the HC. Other studies suggest that familiarity also depends on the HC–EC circuitry [45] , [46] . Our results did show the strongest relationship between hippocampal activity levels and later recollection, as well as high confidence memory scores. Familiarity estimates, on the other hand, did not show any significant correlation with our activity measures. In this study, we focused on the laminar organization of novelty processing and DM effects within the HC–EC circuitry. In principle, a similar approach could be used to assess the functional directionality of memory processing further upstream, focusing for instance on connectivity between PHC, PRC and EC. Given that perirhinal lesions impair familiarity recognition [47] , it is conceivable that a layer-specific organization of novelty responses (and/or DM effects) in these upstream region of the EC would show a relationship to subsequent familiarity rather than recollection. Another functional segregation within the MTL concerns a potential separation of item- and space-related inputs to HC–EC circuitry. Within this scheme, item information from PRC converges to lateral EC, whereas spatial information from PHC converges to medial EC [7] , [48] , [49] . In monkeys, this dissociation appears to be more dominant between posterior and anterior portions of EC [50] . In our study, we displayed images of indoor and outdoor scenes and found strongest activation in PHC and predominantly the medial EC, which is in line with previous findings [51] . However, we note that the most lateral portions of EC were more likely to show fMRI signal dropouts and therefore, we cannot make strong conclusions about functional dissociations between lateral vs medial EC. Furthermore, there is growing evidence for a functional hippocampal specialization along its long axis arising from differences in connectivity and subfield composition between the anterior and posterior HC (for a recent review, see ref. 52 ). Within this functional segregation, the anterior HC has been specifically associated with motivational processing (including novelty), encoding and more global/coarse representations, whereas the posterior HC has been more related to cognition, retrieval and local/detailed representations, respectively. In line with this functional pattern, we found strongest activation during the encoding of novel information in the hippocampal head (anterior HC). However, later recollection, which relates to memory of specific details and fine-grained local representations, was predicted by activation strength in CA1 pyramidal layers in the body of the HC. Regarding novelty-related functional dissociations between HC subfields, reports about the rodent HC have documented increased CA1 pyramidal cell activity during novel experiences (see, for example, refs 23 , 24 ). These results are compatible with computational models according to which CA1 can act as a comparator [25] , [53] , [54] for information stored in CA3/DG (see, for example, ref. 55 ) and direct perforant pathway inputs to CA1, and thereby produces novelty signals. Our results are not inconsistent with these observations and models but do refine them. Indeed, a key aspect of our study is that successfully memorized items are novel items at the time of encoding. Therefore, according to our data the HC receives novelty signals for all new items (signalled via superficial EC) but produces an output from CA1 preferentially for some of them (signalled via pyramidal CA1 and deep EC). Owing to this selectivity, CA1 is not only acting as a generic novelty detector but also generates novelty responses that are tightly linked to successful long-term encoding. These results are compatible with longstanding evidence that generic novelty signals do not require CA1 and can be computed without the HC (for a review see ref. 56 ). For example, novelty signals can be preserved in cases of bilateral hippocampal injury [44] , [57] and extrahippocampal MTL regions can show novelty responses to visual stimuli such as scenes [19] , [20] and in fact compute this very rapidly [58] . Thus our results suggest that selectivity could distinguish hippocampal outputs for novel stimuli from novelty signals at the input level. An internal comparator process as proposed for CA1 (refs 25 , 53 ) could be one mechanism by which such selectivity could be implemented. In our study we differentiated between BOLD activation between pyramidal and apical dendritic layers (SRLM) of CA1. The BOLD contrast in fMRI is an indirect measure of neuronal activity that is based on the changes in deoxyhemoglobin concentration in response to neuronal dynamics at the cellular and microcircuitry level [59] . Simultaneous recordings of local field potentials (LFPs), multi-unit activity and fMRI signals in monkeys [59] have shown that the BOLD response is correlated with postsynaptic LFPs. Importantly, robust BOLD responses can be observed in correlation with LFPs even in the absence of neural spiking [60] . Therefore, it is conceivable that input to the SRLM could cause local BOLD responses that are not associated with a firing response of CA1 pyramidal neurons. Another line of research that combined optogenetic stimulation with fMRI showed that the BOLD response also correlates with neuronal firing of excitatory pyramidal neurons [61] . While there is a controversy whether this relationship is a direct metabolic consequence of firing or rather related to activation of local horizontally spread microcircuits activated by the axons of firing neurons [60] , it is conceivable that firing output of neurons can cause local BOLD responses (either directly or through local horizontal microcircuits). Hence, taken together, it is theoretically plausible that selective BOLD responses can occur in the SRLM and the pyramidal layer of CA1. One interpretational complication to this scenario is that the stratum oriens of CA1 provides input from CA2–CA3 to the pyramidal layer of CA1 (ref. 7 ). Our fMRI measures cannot distinguish to what extent the local BOLD responses associated with the DM effect in the CA1 pyramidal layer are caused by such CA2–CA3 projections. However, our functional connectivity results show that BOLD responses in deep EC are correlated with those in the pyramidal layer of CA1 in the context of the DM-effect, supporting the possibility that DM-related activity of CA1 is indeed related to CA1 output rather than input from CA2–3. To summarize, we show that it is possible to observe layer-specific memory processing in EC and HC non-invasively across the HC–EC circuitry. This approach now paves the way for studies that can incorporate anatomical directionality in addition to measuring activity levels within regions and their correlations across regions. Furthermore, because EC is affected in early stages of Alzheimer’s dementia and the downstream effects of EC pathology are anatomically directed [37] , this approach now can be used to determine which direction of information processing is affected in different stages of the disease. Subjects Twenty-two young subjects (students of the University of Magdeburg, mean age 26±3.6 years, 12 males) participated in the study. Exclusion criteria were metallic implants (other than standard dental implants), tinnitus, known metabolic disorders or a history of neurological or psychiatric disorders. This study was approved by the ethics committee of the University of Magdeburg. All subjects gave written informed consent before participation. Two subjects had to be excluded from further analyses due to strong dropouts in the EC and strong movement artefacts, respectively. Task and design During the fMRI session, subjects performed an incidental visual encoding paradigm. Within one run, 120 new images (60 indoor and 60 outdoor), 60 ‘noise’ images and 60 repetitions of one familiar image were presented randomly. The familiar image and the ‘noise’ images were familiarized using 10 repetitions each directly before the functional MR scan. This also served to familiarize subjects with the task. Subjects made an indoor/outdoor judgment for each image by button press. After a delay interval of about 85 min after starting the fMRI session, subjects performed a recognition memory task on the 120 pictures presented during the fMRI and 60 novel distractor pictures (30 indoor/outdoor). The task was performed outside of the scanner. Subjects rated their confidence of recognition memory on a scale ranging 1–5 (1: ‘sure new’; 2: ‘may be new’; 3: ‘I don’t know whether old or new’; 4: ‘may be old’; 5: ‘sure old’). These confidence ratings were later used as bases for contrast weights in the analysis of the fMRI data and for the calculation of receiver operating characteristics (ROCs) of recognition memory. Stimuli The stimuli consisted of 120 digital photographic images, half indoor and half outdoor scenes, with a size of 500 × 300 pixels and 8-bit grey scales (mean grey value 127±75). Scrambled ‘noise’ pictures were generated by using an 8-bit 50 × 30 pixel random grey value image (same mean and s.d. ), which was upsampled to a resolution of 500 × 300 pixels (without antialiasing or smoothing), resulting in a checkerboard-like image. The fixation target was a black image of the same size with a white fixation star in the middle. The stimuli were projected onto the center of a screen and the participants watched them through a mirror mounted on the head coil, subtending a visual angle of about ±3° by ±2°. Performance indices To assess subjects’ memory performance, we calculated four performance indices from the behavioural data. Recollection and familiarity contributions to memory retrieval were estimated by ROCs. Therefore, a modified ROC curve was fitted to the hit and false alarm rates given by the four possible thresholds from the five ratings. The d’ of this fitted function corresponds to the familiarity estimate, the y axis-offset to the recollection estimate. Furthermore, the corrected hit rate was calculated as third index by subtracting the false alarm rate (response 4/5 for distractors) from the hit rate (response 4/5 for targets). We also computed a high confidence corrected hit rate as a fourth index by only counting the high confidence hits (targets with rating 5) and subtracting only the high confidence false alarms (distractors with rating 5). Please note that the measures recollection and familiarity (estimated by ROCs) are closely related to high confidence corrected hit rate and corrected hit rate, respectively. FMRI data acquisition MRI data were acquired using a 7T MR system (Siemens, Erlangen, Germany). A 32-channel head coil was used (Nova Medical, Willmington, M). Before the fMRI session, a whole-head MPRAGE volume (TE=2.8 ms, TR=2500, ms, TI=1050, ms, flip angle=5°, resolution=0.6 mm isometric; see Fig. 4b ) was acquired. Subsequently, the fMRI encoding session was run. Each subject’s fMRI scan consisted of 370 volumes, each comprising 28 T2*-weighted echo planar slices with a resolution of 0.8 × 0.8 mm (TE=22 ms, TR=2000, ms, slice thickness=0.8 mm, FOV=205 mm, matrix=256 × 256, partial Fourier=5/8, parallel imaging with grappa factor 4, bandwidth=1028 Hz/Px, echo spacing=1.1 ms, echo train length=40, flip angle=90°) in a single session, summing to a session length of ca. 12 min. The slices were acquired in an odd–even interleaved fashion oriented parallel to the HC long axis (see Fig. 2b and Supplementary Fig. 4 for mean EPI images). EPIs were distortion corrected using a point spread function mapping method [62] and motion corrected during the online reconstruction. After that, the high resolution partial structural volume was acquired (T2*-weighted imaging, TE=18.5 ms, TR=680 ms, resolution=0.33 × 0.33 mm, 45 slices, slice thickness=1.5 mm+25% gap, FOV=212 × 179 mm, matrix=640 × 540), with a slice alignment orthogonal to the HC main axis (see Fig. 2a ). Total MRI duration was around 60 min. FMRI data preprocessing and first-level analyses FMRI data pre-processing and statistical modelling were done using ‘SPM8’ (Wellcome Department of Cognitive Neuroscience, University College, London, UK). Raw image data were converted to Nifti images, while preserving the original image parameters. The pre-processing included only slice timing correction (‘unsmoothed data’ used for all ROI-based analyses) and smoothing with two different smoothing kernels: a 1.5- and a 2.4-mm FWHM Gaussian kernel. This was done to analyse activation at group level with high specificity (FWHM<2 × voxel size) and high sensitivity (FWHM=3 × voxel size), respectively. All models were calculated in native space. Encoding-related hemodynamic responses were analysed as a function of subsequent recognition memory success in the recognition memory test by sorting the stimulus onsets according to the five confidence rates. The onsets of the familiar and noise stimuli constituted two additional conditions. Together with the six movement parameters and one ‘error variance’ condition (to take up variance due to invalid responses, that is, failure to press a response button), this resulted in 14 conditions. To assess novelty-related differences in activity, as well as activity changes due to subsequent memory, two types of contrasts were calculated. For ‘novelty’, we contrasted all new images (irrespective of subsequent memory performance) to the familiar images to capture activations due to stimulus novelty. For subsequent memory (difference due to later memory, ‘DM’), we contrasted two positive weights for later recognized stimuli (confidence ratings 4 and 5) and three negative weights of equal value for the later forgotten items (confidence ratings 1, 2 and 3). We classified response category 3 ‘I don’t know whether the image is old or new’ as forgotten because this response category means that a participant does not recognize the repeated item with either familiarity or recollection. Rating 4, ‘may be old’, on the other hand, means that an item is recognized as a repetition. Excluding category 3 from the contrasts would reduce the power of our analyses (comparing group activity maps for both a DM contrast with and without category 3 and found the same regions being activated, but with more power for the DM contrast which includes also the trials for response 3). Please note that the DM contrast includes only the novel items, whose memory was tested afterwards and not the familiar image (which was repeated continuously during encoding). Cross-participant alignment for univariate group analyses To visualize and compare group activity levels in the MTL related with novelty and subsequent memory, we performed cross-participant alignment on a group-specific T1 template by the use of ROI-ANTS [36] . This nonlinear diffeomorphic mapping procedure optimizes regional alignment (based on anatomically defined ROIs) across subjects [63] , [64] . First, the Oxford Centre for fMRI of the brain software library (FSL 5.0.6) was used to register (and reslice) the individual MPRAGE images to the individual mean functional images. This was done with epi_reg, a command-line program that belongs to the FMRI of the Brain’s (FMRIB's) linear registration tool (FLIRT v6.0 (ref. 65 )) and was specifically written to register EPI images to structural images. Second, a study-specific T1 template was created (same resolution as EPIs) in ANTS using the buildparalleltemplate.sh command-line script (cross-correlation similarity metric [66] ). As a result, the study template together with the transformation matrix (from each subject to template space) was obtained. Although these alignment parameters already allow for a good registration to the template, we wanted to further improve normalization for the MTL regions by adding landmarks to the template. Therefore, the hippocampal head (on the first slice on which it appears), EC, hippocampal body and PHC (same slices as hippocampal body) were labelled on the T1 template as landmarks for the subsequent label-guided alignment. Similarly, subject-specific ROIs were adjusted to match the template priors. Third, we applied the expectation-based point set registration (‘pse’; step size: SyN[0.5]) to register the individual MPRAGEs on the T1 template based on the labelled point sets (=MTL masks). The resulting transformation matrix was then applied to each participant’s novelty and DM contrast map, as well as to the MTL masks to verify alignment precision (see Supplementary Fig. 1 ). One subject had to be excluded from the univariate second-level analyses, since the EC regions in particular were improperly registered to the template. Finally, the aligned contrast images of all remaining subjects ( N =19) were submitted to a second-level group analysis in SPM (one-sample t -test). Simulation of type-1 error rates For second-level group statistics, we used our HC/EC template ROI (including the whole HC head and body) as explicit mask since our hypotheses were specifically focused on processing of novel information within the EC-HC circuit. To estimate the probability of false positive clusters, we used the 3dClustSim tool in AFNI ( http://afni.nimh.nih.gov/afni/ ). This program computes the cluster size threshold at chosen values for the alpha significance level and voxel-wise threshold (alpha=Prob(Cluster≥given size)). 3dClustSim requires an estimate of the spatial correlation across voxels, which was determined in SPM for 1.5 and 2.4 mm applied smoothing kernels (FWHM 1.5 mm =2.1 × 2.3 × 1.8 mm 3 and FWHM 2.4 mm =2.9 × 3.2 × 2.4 mm 3 ), respectively. For visualization, second-level result maps were thresholded at P voxel level <0.005 and a cluster size of k 1.5 mm ≥15 voxels and k 2.4 mm ≥25 voxel, respectively. The type-1 error rates of the resulting clusters are listed in Tables 1 and 2 , where all clusters with alpha >0.05 are highlighted (italics). Segmentation of ROIs For each subject, ROIs were manually segmented on the high resolution T2*-weighted images acquired orthogonally to the HC long axis. In parallel, segmentation was verified and adjusted on the MPRAGEs, which had been bias corrected and coregistered to the T2* volumes. The T1-weighted MPRAGE images provided additional information due to their different contrast, lower slice thickness and fewer susceptibility artefacts (especially in the anterior MTL including the EC). Finally, the T2* images and all the ROIs were coregistered and resliced to the individual mean functional EPI images (automatically and/or manually with SPM8). Again all ROIs were checked and (if necessary) corrected to achieve a precise overlay on the functional data (see Fig. 2a for segmentation scheme). ROIs were identified in bilateral hippocampal body, EC, PRC and PHC, which were traced on consecutive coronal slices for each hemisphere separately using MRIcron (Chris Rorden, Version 4, April 2011). Delineation of hippocampal body subfields started anteriorly on the first slice on which the head of the HC was no longer visible (when the uncus disappears). Labelling was continued caudally, ending on the last slice where the inferior and superior colliculi were jointly visible. The HC was segmented into subiculum (Sub), CA1-stratum pyramidale (pyr. CA1; probably also containing portions of the stratum oriens), CA1-SRLM and the remaining portion comprising CA2, CA3 and DG (DG/CA2–3) as shown in Fig. 2a . The CA1/subiculum border was determined by drawing a line perpendicular to the edge of the subiculum touching the medial border of the HC [67] , [68] . Although this marking scheme can result in a small part of the prosubiculum and subiculum proper being counted towards the CA1 subregion, this border was chosen because it could be reliably identified and replicated [68] . Furthermore, this problem of counting portions of subiculum towards CA1 might be especially prominent in the head but is less pronounced in the body (thus the proportion of subiculum being counted towards CA1 is relatively small in comparison with the size of the CA1 ROI). The CA1-SRLM could be distinguished as the hypointense band lying between the more intense DG and CA1-stratum pyramidale cell layers [37] . Voxels overlapping with other ROIs (pyr. CA1, DG/CA2–3) were later deleted from these ROIs and preserved in the SRLM. Finally, CA2, CA3 and DG were marked as one region because there were no reliable borders to discriminate between these structures (DG/CA2–3). The most lateral point of DG (visible due to the SRLM, which appears dark) formed the border between CA1 and DG/CA2–3 and was constructed by drawing a straight, vertical line to the superior border of the HC [67] . Tracing of the EC started anteriorly at the level of the amygdala (if it was not covered by artefacts), moving caudally along the parahippocampal gyrus. As the collateral sulcus ends posteriorly, the posterior EC is winding down as well [14] , merging into the PHC. Laterally, the EC borders the PRC. The opening of the collateral sulcus typically coincides with the lateral border of the EC [14] , and was therefore chosen as lateral limit. Contrary to other markings schemes for the EC, we did not mark the part of the EC within the collateral sulcus that depends on the depth of the collateral sulcus, since this border could not always be reliably assessed due to susceptibility artefacts. The most medial point of the temporal cortex was selected as medial boundary of the EC [68] , which is abutted by the subiculum laterally. Overall, the EC covered ~25 functional (EPI) slices. Artefacts were most frequent in very anterior slices (at the level of the amygdala). Furthermore, dropouts occurred close to the ear canals, primarily affecting the PRC and partially spreading into the lateral EC (ca. 8.5% of EC slices). However, each subject also provided clean EC data. Overall, ~70% of slices covering the EC were usable for the final analysis. Sample EPI slices with and without dropout and are illustrated in the Supplementary Fig. 4 . Furthermore, as artefacts more frequently occurred in the very anterior than posterior and lateral than medial part of the EC, our measurements were preferentially derived from the more posterior EC, covering more medial than lateral EC. Although lateral vs medial or anterior vs posterior portions of the EC might show functional differences due to the differential connections to PHC and PRC as shown in the rat and monkey [7] , [50] , respectively, we did not address this issue here, since further subdivision of the EC layers would have led to very small ROIs. To assess differences in activity between entorhinal regions during novelty processing and successful memory encoding, we divided the EC into three equally sized portions: superficial, middle and deep. Therefore the superficial and deep layers were manually segmented. Although the microscopic anatomical EC layers could not be seen on our T2* images, previous 7T MRI studies of the human EC [13] , [14] have shown that the cytoarchitectural features of EC layers can be distinguished with ultra-high resolution ex-vivo . The cell-dense entorhinal layer II islands, as well as the hypointense lamina dissecans can be robustly observed on MR images with 100 μm isotropic resolution. These studies also show that the superficial third of the human EC mainly covers EC layer II, which gives primarily rise to input into DG and CA3, and probably also includes parts of entorhinal layer III, which projects mainly to the apical dendrites of CA1. In contrast, the deep third of the EC is mostly covered by the deep pyramidal layers V and VI, and is the main target of output from the HC. The middle EC portion, in turn, appears to mainly comprise the cell-free layer lamina dissecans (layer IV following Cajal’s nomenclature) and parts of entorhinal layer III. Furthermore, dendrites of the deep pyramidal neurons might extend into the middle layer and contribute to activation. Regarding this anatomical layering of the EC, our hypotheses focus on the superficial and deep EC regions, which can be relatively clearly assigned to input and output layers, respectively. Functional interpretations about the middle EC section, on the other hand, are uncertain. Thickness of EC ‘layer’ ROIs was about 1–1.5 voxels with respect to the functional resolution (0.8 mm 3 isotropic; see Fig. 2 ). The PRC was defined as the region between the medial and lateral edges of the collateral sulcus (covering medial and lateral banks); the PHC was delineated as the region between subiculum (medial border) and the deepest point of the collateral sulcus. However, PRC and PHC cortices were not the focus of the hypotheses addressed here. In summary, nine ROIs per hemisphere were segmented including the EC (with superficial, middle and deep regions), the subfields/layers of the hippocampal body (pyramidal CA1, SRLM, DG/CA2–3 and Sub), as well as the PHC and PRC. Multivariate Bayes MVB [35] is a multivariate Bayesian decoding scheme in which the presence of a cognitive state is predicted from the distributed activity within a defined ROI. In contrast to classical encoding models like the GLM, MVB makes it possible to compare competing hypotheses about which anatomical structure hosts a particular cognitive process (for a recent application, see ref. 41 ) using individual (not normalized and not smoothed) functional data. This is achieved by constructing and comparing alternative models where different data features (that is, distributed activity in different ROIs) are used in an attempt to explain or predict a particular cognitive process, as specified by a contrast of interest. This model comparison rests on evaluating the relative marginal likelihood (or model evidence) of competing models, approximated using a (negative) free-energy bound [69] . Thus, MVB can be used to decide whether a cognitive state (for example, novelty or subsequent memory) is better explained in terms of activity in one region (for example, superficial EC) than another region (for example, deep EC). Here, using MVB in SPM8 and a sparse-coding prior, we computed log evidences for each subject-specific anatomical mask. We used the unsmoothed functional data to achieve highest anatomical precision. For the second-level (group) analysis, we performed random-effects BMS [39] . Random-effects BMS quantifies the probability that a particular model generated the data for any randomly selected subject, relative to other models, and it is robust to the presence of outliers. The posterior distribution over models is parameterized in terms of a Dirichlet distribution. An intuitive way of comparing posterior model probabilities is by deriving the exceedance probability (xp) of each model, that is, the probability that this model is more probable than any other model tested [39] . Correlating successful encoding with later memory performance Bayesian model comparison showed that within the HC proper/DG, subsequent memory was best explained in terms of activation in pyramidal layers of CA1. In addition, we wanted to test if activation strength in pyramidal layers of CA1 also correlated with later memory performance (across subjects). Therefore, we extracted the effect size (mean contrast estimate for DM) from pyramidal CA1 layers and computed correlations with memory performance. First, we masked each individual (not smoothed and not normalized; Z -transformed) first-level DM activation map with the subject-specific anatomical ROI of pyramidal CA1. Then we calculated the mean contrast estimate across all voxels in our purely anatomically defined mask for each subject. Of note, the DM effect and the behavioural memory measures are not based on the same contrast. The DM effect is calculated by subtracting activation for later forgotten from activation for later recognized scene images. In contrast, the behavioural measures are calculated using false alarms as references. These are responses to scenes that were never presented before (novel distractors in the recognition test), and hence could not have contributed to the DM-effect. Furthermore, the DM-effect is independent of whether the subsequent recognition was high or low confidence. The behavioural memory scores that correlated with DM-related activation, on the other hand, are related to ‘recollection’ and restricted to high confidence ratings (‘high confidence corrected hit rate’) and to an ROC-derived score (‘recollection estimate’). PPI analysis To test if region-specific activation in the EC was functionally correlated with activation of the HC during novelty processing or successful encoding we performed connectivity analyses analogous to the PPI approach. This type of functional connectivity analysis identifies areas having a higher correlation with the time course in a given seed region in one psychological context (for example, novel trials) than in another context (for example, familiar trials). For this analysis, individual superficial and deep EC ROIs were used as anatomical masks (seed region), and the mean time course from all voxels in the specific mask was extracted. The regressors of each subject’s SPM model then comprised the seed time course from the EC region (‘physiological main effect’), the task regressor (‘psychological main effect’: novelty or DM) and the ‘psychophysiological interaction’ vector [70] for assessing condition-dependent interregional coupling (plus the movement regressors as covariates). For the PPI analyses we used the 1.5 mm smoothed EPIs to allow high spatial precision. Finally, we performed cross-participants alignment of the resulting contrast-images using ROI-ANTS to calculate a second-level group activity map. How to cite this article: Maass, A. et al. Laminar activity in the hippocampus and entorhinal cortex related to novelty and episodic encoding. Nat. Commun. 5:5547 doi: 10.1038/ncomms6547 (2014).